Crocodylian diversity peak and extinction in the late Cenozoic of the northern Neotropics Northern South America and South East Asia are today’s hotspots of crocodylian diversity with up to six (mainly alligatorid) and four (mainly crocodylid) living species respectively, of which usually no more than two or three occur sympatrically. In contrast, during the late Miocene, 14 species existed in South America. Here we show a diversity peak in sympatric occurrence of at least seven species, based on detailed stratigraphic sequence sampling and correlation, involving four geological formations from the middle Miocene to the Pliocene, and on the discovery of two new species and a new occurrence. This degree of crocodylian sympatry is unique in the world and shows that at least several members of Alligatoroidea and Gavialoidea coexisted. By the Pliocene, all these species became extinct, and their extinction was probably related to hydrographic changes linked to the Andean uplift. The extant fauna is first recorded with the oldest Crocodylus species from South America. The late Cenozoic of South America included a singular array of animals that lived in isolation from other continents until the formation of the Panamanian Isthmus. This fauna included endemic forms resulting from either vicariance or dispersal events from other continents, such as gavialoid crocodilians now found only in South East Asia [1] . From the Paleogene and Neogene, 26 crocodyliform species are recorded [1] . The high diversity of species in the Miocene of the Amazon region [1] , [2] , the origins of which are yet poorly understood [3] , [4] , [5] , is documented largely in sedimentary basins in Colombia (La Venta), Brazil and Peru (Acre) and Venezuela (Urumaco). In contrast, in modern day ecosystems, overall crocodylian diversity is generally declining and no more than two or three species occur sympatrically [6] , [7] . To be able to ascertain the nature of the crocodylian communities that actually existed requires revisionary taxonomic and stratigraphic work, which has been conducted for the Urumaco sequence [8] , [9] . But how many species lived together and how did these species differ ecologically? Here, we document >50 records of crocodylian remains from 14 localities and show a diversity peak in sympatric occurrence of at least seven species. This degree of crocodylian sympatry is unique in the world and shows that at least several members of Alligatoroidea and Gavialoidea coexisted. Geological context The 50 records of crocodylian remains from 14 localities ( Supplementary Tables S1, S2 ), include two new species, ranging from the middle Miocene Socorro Formation to the early Pliocene [10] San Gregorio Formation ( Supplementary Notes 1 and 2 ). The identification of samples is based solely on cranial material preserving diagnostic features. The stratigraphic sequence correlation of the geological formations ( Fig. 1 , Supplementary Fig. S1–S4 (ref. 10 )) serves to place the localities into a geographic and temporal context. 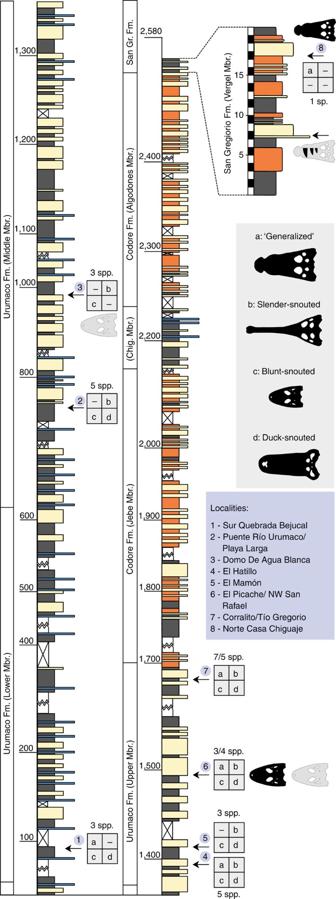Figure 1: Simplified stratigraphic profile of the Miocene and Pliocene of Urumaco. Profile is modified from10, with new data added on San Gregorio Formation. Faunal ecomorphotypes4and number of species are presented for each locality (number above or below gray boxes; note that for locality numbers 6 and 7, two species counts are given; see alsoSupplementary Figs 1–4). Type localities, as well as sites of recovery of referred material, are indicated by black and gray skull outlines respectively. Isolated teeth collected 1 km from type locality (AMU-CURS-302;Supplementary Fig. S10) ofC. falconensismark the earliest re-occurrence of crocodylians in the early Pliocene of Falcón State so far. Gray, mudstone/siltstone/shale; blue, coquinoid limestone; yellow, sandstone; orange, mottled mudstone; white, non-exposure/cover interval. Figure 1: Simplified stratigraphic profile of the Miocene and Pliocene of Urumaco. Profile is modified from [10] , with new data added on San Gregorio Formation. Faunal ecomorphotypes [4] and number of species are presented for each locality (number above or below gray boxes; note that for locality numbers 6 and 7, two species counts are given; see also Supplementary Figs 1–4 ). Type localities, as well as sites of recovery of referred material, are indicated by black and gray skull outlines respectively. Isolated teeth collected 1 km from type locality (AMU-CURS-302; Supplementary Fig. S10 ) of C. falconensis mark the earliest re-occurrence of crocodylians in the early Pliocene of Falcón State so far. Gray, mudstone/siltstone/shale; blue, coquinoid limestone; yellow, sandstone; orange, mottled mudstone; white, non-exposure/cover interval. Full size image Systematic section. Crocodylia Gmelin, 1789Crocodylidae Cuvier, 1807Crocodylinae Cuvier, 1807 Crocodylus falconensis sp. nov. Etymology. After Falcón State, northwestern Venezuela, in which the town Urumaco is situated. Holotype. AMU-CURS-300, an almost complete skull with mandibles ( Fig. 2a–e , Supplementary Fig. S5 ). 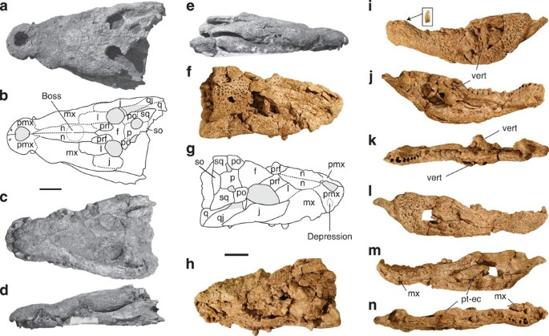Figure 2: Holotypes of new species. (a–e)C. falconensissp. nov. (AMU-CURS-300).f–n)G. brachyrostrisgen. et sp. nov. (AMU-CURS-222). (b,g) Interpretative drawings of skulls. (i–k) Left mandible. Note inset of fourth dentary tooth in (i). (l–n) Right mandible, initially attached to skull. Note that two vertebrae (vert) are fused to the left mandible, and parts of the skull (mx, pt-ec) are fused to the right one. (a,f,k,n) Dorsal, (c,h) ventral, (d) left lateral, (e) right lateral, (i,l) lateral, (j, m) medial views; (f) and (g) were mirror-imaged for clarity. f, frontal; j, jugal; l, lacrimal; mx, maxilla; n, nasal; p, parietal; pmx, premaxilla; po, postorbital; prf, prefrontal; pt-ec, pterygoid and ectopterygoid, q, quadrate; qj, quadratojugal; so, supraoccipital; sq, squamosal; vert, vertebral remains. Scale bar=10.0 cm in (a–e) and 5.0 cm in (f–n). Figure 2: Holotypes of new species. ( a – e ) C. falconensis sp. nov. (AMU-CURS-300). f – n ) G. brachyrostris gen. et sp. nov. (AMU-CURS-222). ( b , g ) Interpretative drawings of skulls. ( i – k ) Left mandible. Note inset of fourth dentary tooth in ( i ). ( l – n ) Right mandible, initially attached to skull. Note that two vertebrae (vert) are fused to the left mandible, and parts of the skull (mx, pt-ec) are fused to the right one. ( a , f , k , n ) Dorsal, ( c , h ) ventral, ( d ) left lateral, ( e ) right lateral, ( i , l ) lateral, ( j, m ) medial views; ( f ) and ( g ) were mirror-imaged for clarity. f, frontal; j, jugal; l, lacrimal; mx, maxilla; n, nasal; p, parietal; pmx, premaxilla; po, postorbital; prf, prefrontal; pt-ec, pterygoid and ectopterygoid, q, quadrate; qj, quadratojugal; so, supraoccipital; sq, squamosal; vert, vertebral remains. Scale bar=10.0 cm in ( a – e ) and 5.0 cm in ( f – n ). Full size image Locality and horizon. Northeastern part of Urumaco, from the early Pliocene San Gregorio Formation (Vergel Member; Norte Casa Chiguaje, locality ‘No. 8’ in Fig. 1 , Supplementary Fig. S2 ), Falcón State. Diagnosis. Medium-sized Crocodylus species with a flattened, broad and robust skull and dentition differing from all other crocodylids in the supraoccipital reaching or almost reaching foramen magnum; orbits and supratemporal fenestrae smaller than in other Crocodylus species at the same ontogenetic stage; premaxillary rostrum expanded, with relatively small external naris, but larger comparatively; premaxillae meet posterior to external naris; nasals excluded from external naris, at least externally; orbits circular and slightly larger than external naris; skull table with shallow depression, extending to the frontal; concave posterior margin of skull roof, no posterior convexity; dorsal surface of rostrum bearing medial dorsal boss; rostrum with dorsoventral constriction posterior to external naris; lateral edges of the palatines between the suborbital fenestrae nearly parallel; anterior-most width of intersuborbital bar wider than posterior-most width.The skull shows obliterated sutures ( Supplementary Fig. S5 ). Size and mass in life was estimated as 4.12 m and 307 kg respectively ( Supplementary Tables S3–S5 ). A medial dorsal boss, a feature shared with other Neotropical Crocodylus species, is well developed. Alligatoridae Gray, 1844 Caimaninae Brochu, 2003 (following Norell, 1988) Globidentosuchus brachyrostris gen. et sp. nov. Etymology. Generic name referring to spherical teeth in posterior part of skull (‘globi’ from Latin globus for sphere; ‘dento’ from Latin dens for tooth; ‘suchus’ after Greek Suchos , in reference to the Egyptian crocodile-headed God Sobek ). Specific name referring to short and wide snout (‘brachy’ from Greek brachys for short; ‘rostris’ from Latin rostrum for snout, in reference to beak-shaped curved prows of Roman ships). Holotype. AMU-CURS-222, an almost complete skull with associated mandibles ( Fig. 2f–n ). Paratype. AMU-CURS-224, fragmentary skull remains associated with mandibles ( Supplementary Fig. S6 ). Referred material. AMU-CURS-223, associated fragmentary cranial and mandibular remains; AMU-CURS-301, posterior part of right mandible with four crushing teeth preserved; AMU-CURS-383 cranium; AMU-CURS-450 isolated mandibular remains (See also Supplementary Fig. S7–S9 ). Locality and horizon. The holotype was collected from El Picache locality (‘No. 6’ in Fig. 1 , Supplementary Fig. S2 ), Cerro José la Paz site, Urumaco Formation (Upper Member), the paratype from Sorongo site at El Picache, the referred material AMU-CURS-223 from an unnamed site at El Picache, AMU-CURS-301 and AMU-CURS-450 from the Domo de Agua Blanca locality (‘No. 3’), Urumaco Formation (Middle Member), and AMU-CURS-383 northwest of San Rafael (‘No. 6’), Urumaco Formation (Upper Member). Diagnosis. Small caimanine species differing from all other crocodylians in having a U-shaped, short and wide skull and deep, robust mandibles; external naris not bisected by nasals; smooth skull surface with weak preorbital ridges but lacking rostral or interorbital ridges; frontal lacks anterior processes and articulates in V-shaped suture with prefrontals rostrally; prefrontals rectangular-shaped, meeting in midline; supraoccipital excludes parietal from posterior skull table edge; dentary and splenial participate in symphysis, which reaches back caudally until seventh mandibular alveolus. Each mandible with 18 teeth; short conical teeth but posterior eight teeth complanate, subspherical and tightly spaced, forming crushing unit; fourth mandibular alveolus is largest, with the largest following dentary alveoli immediately caudal being the whole series from thirteenth alveolus onward; mandible with foramen aërum set in from margin of retroarticular process; articular with laminae both above and below lingual foramen; lingual foramen for articular artery and alveolar nerve perforates surangular/angular suture; surangular pinched off anterior to tip of retroarticular process; surangular–articular suture bowed strongly laterally within glenoid fossa; superior edge of coronoid slopes almost horizontally; splenial forming massive shelf lingual to tooth row; mandibular fenestra large; medial jugal foramen large; margin of orbit flush with skull surface. A strong crushing dentition is developed in a variety of fossil and extant crocodylians, including Caiman brevirostris , Allognathosuchus spp. and Caiman latirostris . None of those taxa, however, develops a crushing unit of the eight posterior-most teeth as is found in G. brachyrostris . The whole series from the thirteenth alveolus (or fourteenth) onward being the largest immediately caudal to the fourth (character 51-1) is unknown in other caimanines, but a feature that G. brachyrostris shares with some globidontan and non-globidontan alligatoroids. G. brachyrostris also shares an angular not extending dorsally beyond the anterior end of foramen intermandibularis caudalis (character 65-1) and the surangular–angular suture lingually meeting the articular dorsal to tip (character 66-1) with most derived caimanines; however, the former occurs independently also in the globidontan Stangerochampsa mccabei . G. brachyrostris shares with Thecachampsa antiqua only an articular bone in which laminae are present both above and below the lingual foramen (character 68-3). A foramen aërum being set in from the margin of retroarticular process (character 70-1) is shared by all Alligatoroidea for which this character is known, but is also present in the crocodyloid Voay robustus . The maxilla broadly separating the ectopterygoid from the maxillary tooth row (character 103-1) is a typical feature of Alligatoroidea (including the new caimanine taxon), but is also found in the outgroup Bernissartia fagesii . Posteriorly flaring lateral edges of the palatine bones that produce a shelf (character 119-1) was found to be shared by most Alligatoroidea with the exception of the basal-most alligatoroid Leidyosuchus canadensis and the globidontan Ceratosuchus burdoshi . A large exposure of the supraoccipital on the dorsal skull table which excludes the parietal from reaching the posterior edge of the table (character 158-3) appears to be plesiomorphic for Caimaninae. Among caimanines, the absence of an anterior process of the frontal, prefrontals contacting medially and a V-shaped frontal-prefrontal suture are features seen also in the fossil and extant Melanosuchus spp. and in the extant Caiman crocodilus . G. brachyrostris differs from Culebrasuchus mesoamericanus in having a curved instead of a linear dentary from d4 to the posterior-most alveolus, a splenial participating in the symphysis, narrower and smaller supratemporal fenestrae with a more pronounced overhang along the medial wall, and a wider more crescent-shaped supraoccipital exposure in dorsal view. It further differs from Centenariosuchus gilmorei in lacking upturned medial orbital margins and in having a larger external mandibular foramen (a smaller foramen is indicated in an angular referred to cf. C. gilmorei ). Caiman brevirostris , another caimanine with crushing dentition [11] , is superficially similar to G. brachyrostris . However, the sutural configuration and shape of the frontals and prefrontals, and the symphyseal participation of the splenial separate both species. The splenial symphysis might be shared with Tsoabichi greenriverensis [12] . The cranial proportions of G. brachyrostris indicate a mean overall size of 1.72 m and body mass of 16.7 kg ( Supplementary Tables S3-S5 ). Alligatoridae Gray, 1844Caimaninae Brochu [4] (following Norell, 1988) Mourasuchus nativus (Gasparini, 1985) Referred material. AMU-CURS-212, a posterior skull roof and braincase ( Fig. 3 ); AMU-CURS-218, additional cranial material. 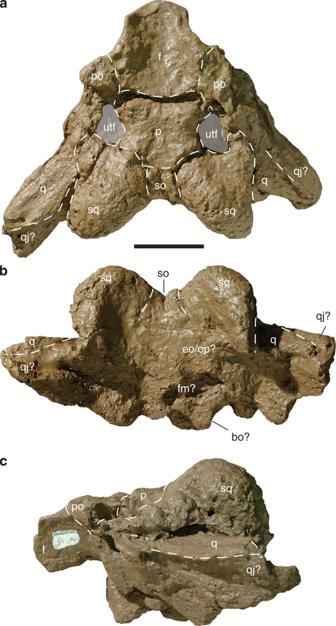Figure 3: Posterior skull roof and braincase ofM. nativus. Specimen (AMU-CURS-212) in (a) dorsal view, (b) occipital view and (c) left lateral view. Note that sutures are generally difficult to trace in occipital and lateral views and that the elements of the braincase floor (for example, basioccipital) shifted laterally towards right. bo, basioccipital; eo/op, exoccipital/opisthotic; f, frontal; fm, foramen magnum; j, jugal; l, lacrimal; mx, maxilla; n, nasal; p, parietal; pmx, premaxilla; po, postorbital; prf, prefrontal; pt-ec, pterygoid and ectopterygoid, q, quadrate; qj, quadratojugal; so, supraoccipital; sq, squamosal; vert, vertebral remains. utf, upper temporal fenestra. Scale bar=5.0 cm. Figure 3: Posterior skull roof and braincase of M. nativus. Specimen (AMU-CURS-212) in ( a ) dorsal view, ( b ) occipital view and ( c ) left lateral view. Note that sutures are generally difficult to trace in occipital and lateral views and that the elements of the braincase floor (for example, basioccipital) shifted laterally towards right. bo, basioccipital; eo/op, exoccipital/opisthotic; f, frontal; fm, foramen magnum; j, jugal; l, lacrimal; mx, maxilla; n, nasal; p, parietal; pmx, premaxilla; po, postorbital; prf, prefrontal; pt-ec, pterygoid and ectopterygoid, q, quadrate; qj, quadratojugal; so, supraoccipital; sq, squamosal; vert, vertebral remains. utf, upper temporal fenestra. Scale bar=5.0 cm. Full size image Locality and horizon. AMU-CURS-212 was collected from El Mamón locality, Upper Member of the Urumaco Formation (‘No. 5′ in Fig. 1 , Supplementary Fig. S2 ) and AMU-CURS-218 from Puente Río Urumaco locality, Middle Member of the Urumaco Formation (‘No. 2’ in Fig. 1 , Supplementary Fig. S2 ). Diagnosis. M. nativus is the second species of duck-snouted (‘nettosuchid’) caimanines, besides M. arendsi [13] , and is the fourteenth crocodylian recognized from the Neogene (that is, Urumaco Formation) of Urumaco ( Fig. 4 ). Especially AMU-CURS-212 preserves enough of the diagnostic features (that is, small crest in midline of parietal; entire posterior part of skull table raised; squamosals particularly high and strongly developed forming transverse ridge) for species recognition [14] , [15] . Previously recognized from the Ituzaingó fauna in Argentina, and Acre in Brazil [1] , [15] , [16] , the palaeogeographic occurrence of the species was thus spanning >4000, km from the Buenos Aires region in the South to the Caribbean Sea in the North, which is more than any of the living crocodylians does in South America today. 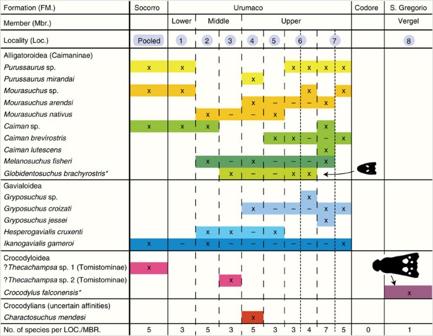Figure 4: Taxic crocodylian diversity and locality data. New described taxa are indicated by asterisk and images scaled to same size. Locality numbers in circles correspond to locality names given inFig. 1. Notice that the total number of species does not count reconstructed records in the middle of stratigraphic extremes of distribution. Figure 4: Taxic crocodylian diversity and locality data. New described taxa are indicated by asterisk and images scaled to same size. Locality numbers in circles correspond to locality names given in Fig. 1 . Notice that the total number of species does not count reconstructed records in the middle of stratigraphic extremes of distribution. Full size image Phylogenetic analysis The phylogenetic analysis including the new Crocodylus species recovered only one most parsimonious tree (MPT; length=59, CI=0.6 and RI=0.7; see Fig. 5a ). As in previous analyses [17] , [18] , the crown Crocodylus was monophyletic. C. palaeindicus is sister taxon of the crown clade, but support is weak. The New World assemblage represents a monophyletic and well-supported clade, having C. falconensis sp. nov. as the basal-most representative species and the sister group of a clade comprising the extant species (see also Supplementary Fig. S10 for additional crocodylian teeth from the San Gregorio Formation). The New World crocodiles are supported by two unambiguous synapomorphies: the dorsal surface of rostrum bears medial dorsal boss (15-1) and the palatine–pterygoid suture lies nearly at the posterior angle of suborbital fenestra (20-0). These characters seem to have evolved shortly after the dispersion event from the Old World to the New World [19] , as they are present in C. falconensis sp. nov. already early in the Pliocene. Some features are present in all extant species of the clade, but due to the incompleteness of C. falconensis sp. nov., they could not be traced back to the early evolution of the group: ventral tubercle of proatlas more than one-half the width of the dorsal crest (1-0), and the pterygoid surface lateral and anterior to internal choana is pushed inward around choana to form the “neck” surrounding aperture (22-2). These are unknown in C. falconensis sp. nov., and may represent synapomorphies of the New World crocodiles or only of the extant species. Nevertheless, some features were recovered as unambiguous synapomorphies of the extant group: the posterior margin of the skull roof with a posterior process, forming a distinct convexity (30-1), and the posterior process of palatines have nearly parallel sides (31-1). C. acutus and C. intermedius share an anterior process of palatines wider than the posterior process (32-2). Although only one feature groups them together, the sister-group relationship between C. acutus and C. intermedius has been already proposed by molecular phylogenies [7] , [19] , [20] , [21] . The New World clade is a well-supported group and has accumulated distinctive differences from its sister taxon, C. niloticus , and other extant and extinct crocodile species ( Fig. 5a ). 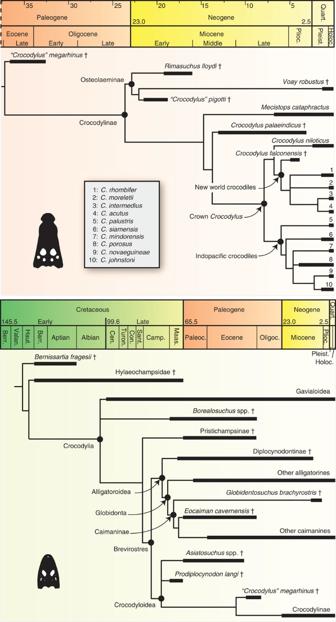Figure 5: Simplified phylogenetic hypotheses and stratigraphic occurrences of new taxa. The occurrence and placement22,24of the two new species is indicated based on analyses outlined inSupplementary notes. Figure 5: Simplified phylogenetic hypotheses and stratigraphic occurrences of new taxa. The occurrence and placement [22] , [24] of the two new species is indicated based on analyses outlined in Supplementary notes . Full size image The phylogenetic analysis including G. brachyrostris gen. et sp. nov. resulted in a total of 20,160 most parsimonious trees (minimum length=650; Fig. 5b ). The computed strict consensus was overall in accordance with the one recovered by Brochu et al . [22] , including all major monophyletic groups, but differing slightly in relationships among highly nested gavialids and tomistomine crocodyloids ( Supplementary Fig. S11, S12 ). Relationships within Caimaninae are also as in Brochu et al . [22] , with G. brachyrostris gen. et sp. nov. being sister to all remaining caimanine species. Character (66-1; surangular–angular suture lingually meets articular dorsal to tip) was revealed as a potential unambiguous and unequivocal synapomorphy of Caimaninae. The phylogenetic analysis recovered C. falconensis sp. nov. as sister taxon to all remaining New World Crocodylus species ( Fig. 5a ), suggesting that tropical South America was probably the center of origin of the Crocodylus neotropical radiation, after transatlantic dispersal either across the Atlantic from Africa or across the Pacific from Asia [23] . All living species of Crocodylus last shared a common ancestor within the past 15 million years, with the group first appearing in the Old World [17] . The monophyly of the New World clade ( C. falconensis +extant neotropical species) and its minimal early Pliocene age is supported, which has been estimated from both the fossil record and molecular markers [7] , [17] , [24] . The analysis with G. brachyrostris gen. et sp. nov. supports the monophyly of Caimaninae [12] ( Fig. 5b ) and a close relation between Tsoabichi greenriverensis and extant dwarf caimans ( Supplementary Fig. S11 ). Globidentosuchus is at the stem of the caiman lineage, representing the sister taxon to all remaining caimanines, including the hitherto basal-most Eocaiman cavernensis (Paleogene, South America) [12] . Adding one of the oldest caimanines known, Necrosuchus ionensis (early Paleocene, Argentina), did not change the basal-most position of Globidentosuchus , but reduced overall resolution among basal caimanines ( Supplementary Fig. S12 ). As such, Globidentosuchus provides insights into character evolution and polarity (for example, symphyseal shortening that led to exclusion of splenial; large exposure of supraoccipital on skull table), and represents an example of the preservation of basal species in the tropics [25] . Recently, a report of two new caimanines, one basal form from the early Miocene Culebra Formation ( C. mesoamericanus ) and a more highly nested form from the early or middle Miocene Cucaracha Formation ( Centenariosuchus gilmorei ) of Panama was presented [25] . C. mesoamericanus shares with Globidentosuchus , for example, a large exposure of the supraoccipital on the posterior skull roof, but differs in the anterior extent of the splenial, with a termination before the symphysis and larger supratemporal fenestrae without a large overhang being present in the Panamanian taxon. The presence of yet another basal form greatly underscores the importance of the Central American and Northern South American region for the evolution of the whole clade. The extreme ecomorphological breadth among the Urumaco crocodylians with at least seven sympatric species ( Fig. 4 ), ranging from small, blunt-snouted ‘crushers’ with body sizes and masses ranging from 1.5–2 m and 10–820 kg (for example, Globidentosuchus , Supplementary Tables S3–S5 ) to several giant-sized forms, clearly suggests niche partitioning [5] , [26] . The duck-snouted Mourasuchus is represented by two species, with our discovery of M. nativus for Urumaco. The gavialoid Gryposuchus and the ‘generalist’ Purussaurus reached 8–11.5 m and 1.7–3.5 t [8] , [9] and overlap with or exceed some of the other largest crocodyliforms known, such as the pholidosaurid Sarcosuchus (Cretaceous, Africa) and alligatoroid Deinosuchus (Cretaceous, North America), the tomistomine Rhamphosuchus (Miocene, Indian subcontinent), and C. thorbjarnarsoni (Plio–Pleistocene, Kenya) [24] , [27] , [28] . The crocodylian disparity is indicative also of food web complexity, with the smaller to medium size species acting as meso-predators and the giant Gryposuchus and Purussaurus as apex predators in the system [2] , [9] . In modern South American assemblages the lower size spectrum is covered by dwarf caimans ( Paleosuchus ), whereas the upper end remains devoid, with the largest living South American crocodylian, the black caiman ( Melanosuchus niger ), reaching usually no more than 4.5 m (ref. 6 ). The disparity encountered among Urumaco crocodylians appears to be rivaled by fossil crocodylomorph faunas from Eocene localities (for example, middle Eocene Bridger and lower Eocene Green River Formations in Wyoming; the World Heritage site of Messel, a Konservatlagerstätte near Darmstadt, Germany) and the Late Cretaceous crocodyliform assemblage from the Maevarano Formation of Madagascar [29] . The North American formations however crop out over huge areas and although morphological and dietary disparity is apparently high [30] , the actual level of sympatry of taxa, was not [31] , [32] . In the Maevarano Formation, which crops out in northern Madagascar yielding an astounding array of vertebrates including dinosaurs, levels of sympatry are also high, although including largely crocodylomorph taxa [26] rather than members of crown Crocodylia. In contrast, the European Messel locality is fairly restricted in exposure. Of the seven taxa currently recognized in Messel only Asiatosuchus and Diplocynodon species are common, indicating that they were true lake inhabitants—the other taxa were washed in only occasionally from adjacent habitats [33] . In general, the size and mass spectrum of the Eocene taxa from Messel is also more restricted compared with that of the Urumaco fauna, ranging between 0.8 and 5.0 m in length. In contrast, the sampling of the Miocene crocodylians in Urumaco was done mainly by surface collecting in relatively restricted localities ( Supplementary Fig. S1 ). The lithology and depositional environment of the fossil-bearing sediments in each locality is interpreted as preserving fossils in situ or with very little transport. It is thus reasonable to assume sympatry of the species, which were recovered in each of the localities. The new stratigraphical and geographical information presented, together with specific references to numerous specimens in collections and their identifications, leaves no doubt about the sympatry of species reported in this paper. The disarticulated nature of the fossils we find in the field in Urumaco, does not preclude the same stratigraphical origin and contemporaneity, from strata well documented in the new or synthesized geological information presented in this paper. Furthermore, in most cases, many skeletal materials of the same individual are found in association, and never together with remains of other individuals, showing thus that post-mortem transport does not result in spurious associations of species in a site. Representatives of Alligatoroidea, especially Caimaninae, and Gavialoidea, constitute the highest percentage of species in the Urumaco Formation (and the underlying Socorro Formation; Fig. 4 ). In the case of the material tentatively referred to Thecachampsa and Charactosuchus (‘ Brasilosuchus ’) mendesi , a systematic assignment is less clear. Previous works have identified the former pertaining to Crocodylidae [34] , [35] or Crocodyloidea [2] , and the latter to either Crocodylidae [1] , Gavialoidea [2] or Gavialidae [34] , [35] , [36] . In the case of C. mendesi , although no ‘non-crocodylian’ taxa have been so far recovered from post-Middle Miocene rocks, incompleteness of the fossil material currently restricts an assignment beyond Crocodyliformes incertae sedis [37] . On the other hand the Thecachampsa material is regarded as belonging to Tomistominae, which according to anatomical, fossil and developmental data (but contra molecular data) are within Crocodylidae [38] ( see Supplementary Note 3 ). Our results further revealed that disparity is high (for example, indicated by the presence of ecomorphotypes, Fig. 1 ) throughout most localities studied and at least in three out of the seven localities within the Urumaco Formation (nos. 4, 6 and 7), all four ecomorphotypes are present prior to the drastic faunal turnover. Palaeoenvironmental reconstructions based on palynofloras from the Urumaco Formation suggest a continuation of the Amazonian forest into northwestern Venezuela during the Miocene [39] , with the faunal context including marginal marine, freshwater and continental vertebrates [40] . The latest Miocene-early Pliocene Codore Formation flora replaced the Amazonian palynoflora with xerophyte-dominated vegetations during the major environmental change related to the collapse of the Urumaco delta in the late Miocene, which correlates with a major uplift of the northern Andes [41] and the eastward changing hydrograph course of a paleo-Orinoco River [10] , [42] . From the El Jebe Member, Codore Formation, faunal elements such as glyptodontids [43] and grassy wetlands ciconiid birds [44] were recovered. These discoveries suggest that the absence of crocodylians from the Codore Formation ( Fig. 4 ) is not a sampling bias. Temperature is usually one of the main parameters limiting crocodylian distribution patterns [3] . The overlying Pliocene San Gregorio Formation, however, represents sedimentary accumulation in alluvial fans ( Fig. 1 and Supplementary Fig. S4 ) [10] , and the aquatic paleoenvironment is reconstructed as a tropical wetland with meandering channels and inundate savanna [25] . Therefore, the turnover was clearly not driven by temperature changes, as the mean annual range values in the Caribbean did not vary significantly until the upper Pliocene [45] . Instead, the lack of the diverse crocodylian fauna previously present in the region during the Miocene clearly shows the turnover to a new community was most likely coupled with the documented climatic and hydrographic changes linked to the Andean uplift [10] , [41] , [42] . Phylogenetic framework To elucidate the phylogenetic position of the new described species within Crocodylia, two separate maximum parsimony analyses were performed using TNT v. 1.1 (ref. 46 ) (see Supplementary Fig. S11 and S12 ; Supplementary Note 3 ). The first analysis including C. falconensis sp. nov. is based on a matrix of 32 morphological characters, coding 29 characters that vary inside Crocodylinae, and adding two new characters. An exhaustive branch-and-bound search strategy was conducted performing the “implicit enumeration” option. For the second analysis G. brachyrostris gen. et sp. nov. and Necrosuchus ionensis were added to the 179-characters matrix of Brochu et al . [22] , which included 95 ingroup taxa and Bernissartia fagesii as outgroup. For these analyses, a heuristic search (traditional search; space for 50,000 trees in memory, random seed=1) with 1,000 random additional sequence replicates with 100 trees saved per replication and tree-bisection reconnection option was performed. In all analyses, characters were set as non-additive. Length and mass estimation Estimating the length and mass of the newly described taxa ( Supplementary Tables S3–S5 ) followed previously published linear regression formulas of Webb and Messel [47] , which have been used also on fossil taxa [27] , [48] , as well as those used by Hurlburt et al . [49] and Platt et al . [50] , [51] . Hall et al . [52] indicated that there is a discrepancy of 4% among dorsal cranial length measurements between freshly killed animals and dried and cleaned skulls of C. novaeguineae [53] . As such, the size and mass estimates herein are treated as conservative underestimates of real size. In the case of applying the regressions of Hurlburt et al . [49] to Globidentosuchus , the orbito-cranial length-based value led to an estimated total length of more than 3 m, which we treat here as a strong overestimation. We nevertheless kept the values in addition to the other results in Supplementary Table S3 and the body mass estimates in Supplementary Table S5 , but marked them with an asterisk and put them in square brackets. Note that in-depth osteological description of both new species is in preparation elsewhere. Nomenclatural acts This published work and the nomenclatural act it contains have been registered in ZooBank, the proposed online registration system for the International Code of Zoological Nomenclature (ICZN). The ZooBank LSIDs (Life Science Identifiers) can be resolved and the associated information viewed through any standard web browser by appending the LSID to the prefix ‘ http://zoobank.org/ ’. The LSID for this publication is: urn:lsid:zoobank.org:pub:E4D47A14-9D74-40B9-8B19-ABA141C8AE1E. How to cite this article: Scheyer, T. M. et al . Crocodylian diversity peak and extinction in the late Cenozoic of the northern Neotropics. Nat. Commun. 4:1907 doi: 10.1038/ncomms2940 (2013).